The effects of carbon dioxide and temperature on microRNA expression inArabidopsisdevelopment Elevated levels of CO 2 and temperature can both affect plant growth and development, but the signalling pathways regulating these processes are still obscure. MicroRNAs function to silence gene expression, and environmental stresses can alter their expressions. Here we identify, using the small RNA-sequencing method, microRNAs that change significantly in expression by either doubling the atmospheric CO 2 concentration or by increasing temperature 3–6 °C. Notably, nearly all CO 2 -influenced microRNAs are affected inversely by elevated temperature. Using the RNA-sequencing method, we determine strongly correlated expression changes between miR156/157 and miR172, and their target transcription factors under elevated CO 2 concentration. Similar correlations are also found for microRNAs acting in auxin-signalling, stress responses and potential cell wall carbohydrate synthesis. Our results demonstrate that both CO 2 and temperature alter microRNA expression to affect Arabidopsis growth and development, and miR156/157- and miR172-regulated transcriptional network might underlie the onset of early flowering induced by increasing CO 2 . According to the Intergovernmental Panel on Climate Change (IPCC 2007) (ref. 1 ), atmospheric CO 2 concentration will raise from 389 parts per million (p.p.m.) in 2005 to 550–700 p.p.m. by 2050 and to 650–1,200 p.p.m. by 2100, which will result in a global climatic warming of 1.1 to 6.4 o C by the end of this century. CO 2 is a major component in photosynthetic reaction that converts solar energy into energy stored in carbohydrates, therefore, controlling plant yield. Elevated [CO 2 ] raises photosynthetic rate and plant primary net production or biomass [2] , while rising temperature increases the ratio of photorespiratory loss of carbon to photosynthetic gain, thus having an opposite effect [3] . In Arabidopsis , elevated atmospheric [CO 2 ] enhances photosynthetic rate, and reduces stomatal density and conductance, resulting in a higher amount of plant mass and seeds [4] , while mildly increased temperatures leads to fewer rosette leaves [5] and lengthened hypocotyls [6] . Mildly elevated temperature can also act as a potent inducer of early flowering in Arabidopsis [5] ; by contrast, elevated [CO 2 ] can advance [4] , [7] , delay [8] , [9] , or impose no change [10] on Arabidopsis flowering time, depending on plant ecotypes, genotypes and growing conditions [7] . Auxin has a critical role in regulating cell elongation, division and differentiation during plant growth, and is known as plant ‘nervous system’ in mediating plant responses to environmental changes. Elevated [CO 2 ] can affect root hair development through auxin signalling [11] , while mildly increased temperature promotes auxin-mediated hypocotyl elongation in Arabidopsis [6] . Both elevated [CO 2 ] and elevated temperature have been shown to affect gene expressions. It was demonstrated that a high level of [CO 2 ] altered the expression of the genes involved in regulating flowering time [12] , carbon accumulation, defence, redox control, transport, signalling, transcription and chromatin remodelling in Arabidopsis [13] . It can also modify gene expression in Populus [14] , sugarcane [15] , Chlamydomonas reinhardtii [16] and soybean [17] . Similarly, a mild increase of 2–4 °C above the optimum 23 °C affected the expression of a significant number of genes, including splicing regulatory genes, and several robust early markers for flower development [4] . Non-coding small RNAs (smRNAs) of 21–24 nucleotides (nts) function as important regulators of gene expression in nearly all eukaryotes [18] . SmRNAs consist predominantly of microRNAs (miRNAs) and small interfering RNAs (siRNAs). The primary function of the former is to silence genes by forming a complex with Argonaute (AGO) family proteins to guide sequence-specific cleavage of messenger RNAs (mRNAs) or to repress their translation, while the latter may target mRNAs and also mediate siRNA-directed DNA methylation (RdDM) [18] . SmRNAs recognize targets by Watson–Crick base pairing to transcripts to specify the identities of the genes to be silenced [18] . Both biotic and abiotic stresses have been shown to alter the expressions of plant miRNAs, and also generate new miRNAs [19] . For example, freezing (0 °C) (ref. 20 ), low (4 °C) (ref. 21 ) and ambient (16 °C) (ref. 22 ) temperatures have been demonstrated to alter the expressions of mostly different miRNAs. In this study, we identify the significant expression changes in known and predicted miRNAs that are regulated by doubling the amount of atmospheric [CO 2 ] or increasing 3–5 °C temperature. We also detect inversely correlated expression changes in the target transcripts of these miRNAs that are involved in regulating flowering time, auxin-signalling, stress responses and potential cell wall carbohydrate syntheses. Our results suggest that a long-term elevated [CO 2 ] and elevated temperature affect plant development and growth through miRNAs, and provide potentially a miRNA regulatory mechanism for CO 2 -mediated flowering time change. Known miRNAs regulated differentially by CO 2 and temperature We grew Arabidopsis plants with [CO 2 ] as the only variant (430 p.p.m. as the control, and 810 p.p.m. as the testing condition), or with temperature as the only variant (22±0.5 o C as the control, and 28±0.5 o C as the testing temperature) in well-controlled environments (see Methods). Total RNAs were isolated from uppermost fully expanded rosette leaves of CO 2 - and temperature-treated plants before or at early bolting stages ( Fig. 1 ) and used to make smRNA-seq libraries (Methods). These leaves have the largest surface areas for photosynthesis, and are easy to be collected according to specific developmental phenotypes ( Fig. 1 ; Methods). Six to eight million sequence reads were obtained from sequencing these libraries ( Supplementary Table S1 ). The read length distribution analysis revealed that reads mapped to genome were enriched with 20–24 nt reads, and the most abundant among them were 21 and 24 nt, which represent the lengths of the majority of miRNAs and siRNAs, respectively ( Supplementary Fig. S1 ). 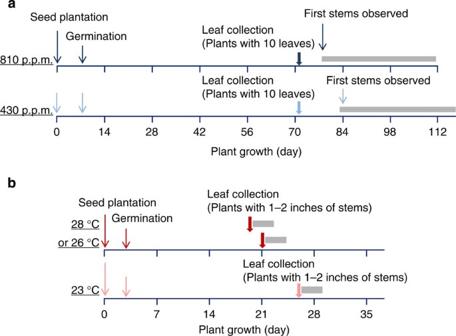Figure 1: Elevated CO2and temperature promoteArabidopsisflowering. Presented areArabidopsisplant growing periods starting from seed plantation to flowering time under (a) 430 and 810 p.p.m. [CO2] and (b) 23 °C and 26 °C or 28 °C temperatures. Big arrows indicate the time when leaf samples were collected. Uppermost fully expanded leaves were collected from 10 leaves stageArabidopsisplants grown under different CO2concentrations before bolting stage or from plants with 1–2 inches of stems grown under different temperatures at the early bolting stage. Dark blue: 810 p.p.m.; light blue: 430 p.p.m.; red: 26 °C or 28 °C; pink: 23 °C; grey rectangles: the period of time when plant flowerings onset. After obtaining miRNA sequence expression levels ( Supplementary Table S1 ), miRNAs including isomirs and miR-siblings altered significantly by elevated [CO 2 ] or elevated temperature were determined ( Table 1 , ; Fig. 2 ; Supplementary Tables S2–S7 ; Supplementary Note 1 ). For miRNA families containing differentially regulated miRNAs, expression changes were calculated for each individual member, as well as for the whole family, and statistical significances were found in all families ( Supplementary Data 1–4 ). Figure 1: Elevated CO 2 and temperature promote Arabidopsis flowering. Presented are Arabidopsis plant growing periods starting from seed plantation to flowering time under ( a ) 430 and 810 p.p.m. [CO 2 ] and ( b ) 23 °C and 26 °C or 28 °C temperatures. Big arrows indicate the time when leaf samples were collected. Uppermost fully expanded leaves were collected from 10 leaves stage Arabidopsis plants grown under different CO 2 concentrations before bolting stage or from plants with 1–2 inches of stems grown under different temperatures at the early bolting stage. Dark blue: 810 p.p.m. ; light blue: 430 p.p.m. ; red: 26 °C or 28 °C; pink: 23 °C; grey rectangles: the period of time when plant flowerings onset. Full size image Table 1 A summary of miRNA analyses. 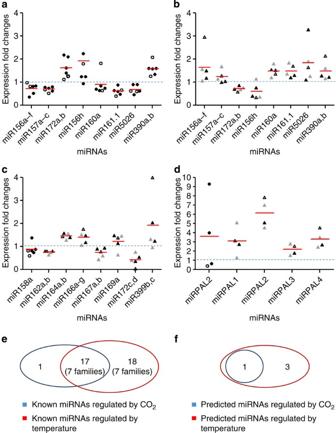Figure 2: MiRNAs differentially regulated by elevated CO2and temperatures. Presented are expression fold changes in known miRNAs regulated by both (a) elevated [CO2] and (b) elevated temperature and (c), elevated [CO2] or elevated temperature specifically, and in (d), predicted miRNAs that are differentially expressed under these two conditions. MiRNA fold changes were calculated by 810 p.p.m.-over 430 p.p.m.-, 28 °C-over 22 °C- or 23 °C-, or 26 °C-over 23 °C-treated samples. The overlapping oval shapes indicate the numbers of miRNAs that were regulated by (e) temperatures and (f), CO2conditions. Empty circles: fold changes of miRNA sequence reads between different [CO2]-treated samples. Solid circles: expression fold changes between different [CO2]-treated samples determined by stem-loop RT–qPCR. Empty triangles: fold changes of miRNA sequence reads between different temperature-treated samples. Grey and solid triangles: miRNA expression fold changes between the samples treated by different temperatures, 26 °C over 23 °C and 28 °C over 23 °C, respectively, determined by stem-loop RT–qPCR. The statistical tests were performed to obtain fold changes of sequence reads usingχ2-test (P<0.01), and Benjamini-Hochberg method for multiple-testing correct (q<0.05). Full size table Table 2 Predicted miRNAs and their function description. Full size table Figure 2: MiRNAs differentially regulated by elevated CO 2 and temperatures. Presented are expression fold changes in known miRNAs regulated by both ( a ) elevated [CO 2 ] and ( b ) elevated temperature and ( c ), elevated [CO 2 ] or elevated temperature specifically, and in ( d ), predicted miRNAs that are differentially expressed under these two conditions. MiRNA fold changes were calculated by 810 p.p.m.-over 430 p.p.m.-, 28 °C-over 22 °C- or 23 °C-, or 26 °C-over 23 °C-treated samples. The overlapping oval shapes indicate the numbers of miRNAs that were regulated by ( e ) temperatures and ( f ), CO 2 conditions. Empty circles: fold changes of miRNA sequence reads between different [CO 2 ]-treated samples. Solid circles: expression fold changes between different [CO 2 ]-treated samples determined by stem-loop RT–qPCR. Empty triangles: fold changes of miRNA sequence reads between different temperature-treated samples. Grey and solid triangles: miRNA expression fold changes between the samples treated by different temperatures, 26 °C over 23 °C and 28 °C over 23 °C, respectively, determined by stem-loop RT–qPCR. The statistical tests were performed to obtain fold changes of sequence reads using χ 2 -test ( P <0.01), and Benjamini-Hochberg method for multiple-testing correct ( q <0.05). Full size image We verified some differentially regulated miRNAs in four pairs of independently grown plant samples using commercially available Taqman MicroRNA Assays (Invitrogen Inc.). These assays were developed for quantifying specific Arabidopsis miRNAs based on a stem-loop reverse transcriptase quantitative PCR (RT–qPCR) method [23] . Seventeen miRNAs from seven families including miR156a–f, −156h, −157a–c, −160, −161.1, −172a, b, −390a, b and −5026 were verified to be regulated by both CO 2 and temperature, and all except miR390a, b were altered inversely by these two conditions ( Table 1 ; Fig. 2a,b,e ; Supplementary Data 5, 6 ). An additional 18 miRNAs from seven families were affected only by elevated temperature, including miR162a, b, −164a, b, −166a-g, −167a, b, −169a, −172c, d and −399b, c ( Table 1 ; Fig. 2c ; Supplementary Data 6 ); miR158a expression was changed significantly only by elevated [CO 2 ] ( Table 1 ; Fig. 2c ; Supplementary Data 5 ). RT–qPCR products were shown as correct sizes in agarose gels ( Supplementary Fig. S4 ). For each verified miRNA, the same expression trend was shown in four biological replicates for all CO 2 -regulated miRNAs, except miR156h and miR158a in three replicates ( Fig. 2a ; Supplementary Data 5 ). Both 26 and 28 °C (23 °C as control) grown samples were analysed because Arabidopsis plants displayed similar phenotypes at both temperatures ( Fig. 1 ), although to a lesser extent at 26 °C. The same expression trend was detected four times for all miRNAs except miR156h, −157, −169a and −399b, c three times ( Fig. 2b,c ; Supplementary Data 6 ). For each miRNA, the same expression trend shown at least four times in all experiments is statistically significant ( Supplementary Methods ). Prediction and expression analysis of new miRNAs Our computational analysis has led to the prediction of 59 new miRNAs ( Table 1 ; Supplementary Figs S2 and S3 ; Supplementary Data 7–9 ) using miRCat [24] and a plant-specific miRDeep methods ( Supplementary Methods ) [25] , [26] . To validate these newly predicted miRNAs, we compared mature miRNA sequences to smRNAs that were co-precipitated in AGO protein complexes by AGO antibodies [27] , and identified 26 miRNAs preferentially associated with AGO1, and eight equally with both AGO1 and AGO4 ( Supplementary Data 10 ). These are more likely to be miRNAs because miRNAs are preferentially bound to AGO1, while siRNAs to AGO4 (ref. 27 ). Among them, 10 were mapped to precursors in miRBase18, but differed from annotated mature miRNA sequences ( Supplementary Data 11 ). Furthermore, 16 miRNAs were found to have messenger RNA cleavage products in Degradome-seq database [28] ( Supplementary Methods ; Supplementary Note 2 ; Supplementary Data 7 ). Transcripts of 44 precursors were also detected in RNA-sequencing datasets (RNA-seq; Supplementary Data 7 ). Fifty-four predicted mature miRNAs were found to be conserved with the genomes of other plant species with two mismatches at most ( Supplementary Data 12 ). Among all predicted miRNAs, four were increased significantly by elevated temperature, and one decreased by elevated [CO 2 ] ( Fig. 2d,f ; Table 1 ). Their target genes and annotated functions are described in Table 2 . These expressions were further confirmed in RT–qPCR experiments in three biological replicates except miRPAL2, which was both up- and downregulated by elevated [CO 2 ] ( Fig. 2d ; Supplementary Data 13,14 ). The expressions of the target transcripts of miRNAs As most miRNAs cleave their target transcripts to suppress their function, we thus performed RNA-seq experiments to determine whether differentially regulated miRNAs can lead to inversed expression changes in their target transcripts. Three pairs of biological replicates were sequenced for each pair of growing condition; one pair of libraries were generated from the same total RNA samples that were used to make the smRNA-seq libraries (see Methods). Twenty-six to forty-nine million raw reads were obtained from sequencing these libraries. Computational analyses led to the identification of differentially expressed mRNAs regulated by elevated [CO 2 ] or/and elevated temperature ( Supplementary Table S8 ; Supplementary Data 15,16 ). 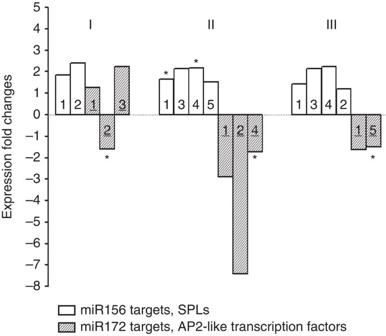Figure 3: The expressions in miR156 and miR172 targets regulated by CO2. Presented are CO2-regulated expression fold changes in miR156/157 and miR172 target transcripts of genes encodingSPLs andAP2-like transcription factors in three biological replicates, I, II, and III. The expression changes inSPLs andAP2-like transcription factors were identified in RNA-seq experiments. Bars without colour representSPLs; numbers on these bars, 1, 2, 3, 4 and 5 representSPL10, SPL9, SPL13A, SPL13B and SPL2. Bars in grey colour representAP2-like transcription factors; numbers on the bars, 1, 2, 3, 4 and 5 areTOE1, SMZ, TOE3, TOE2, andSNZ, respectively. The statistical tests were performed on transcript fold changes using Student’st-test by comparing fragments per kilobase of transcript per million mapped reads or FPKM value (sample size) between samples, and the numbers are shown inTable 3. Fold changes in target transcripts are statistically significant withP<0.01 (FDR test:q<0.1), orP<0.03 (FDR test: 0.1<q<0.2, marked by *). Expression correlations between differentially regulated miRNAs and their target transcripts were thus identified ( Table 3 ). These miRNAs include miR156a–f/157a–c, −172a–d, −160a, −164a, b and a predicted miRPAL2 regulated by CO 2 and temperature, miR169a and miR399b, c by elevated [CO 2 ] only, and miR162a, b by elevated temperature only ( Table 3 ; Supplementary Table S8 ). Table 3 A summary of the expression trends of miRNAs and their target transcripts. Full size table Elevated CO 2 affects the miR156-regulated flowering pathway In this study, we showed that miR156 and miR157 decreased, and miR172 increased in expression significantly under elevated [CO 2 ]. The downregulations of miR156/157 expressions correlated with upregulations of several squamosa promoter binding protein-like ( SPLs ) gene transcripts; these SPLs include SPL10 in all three biological replicates, SPL13A and SPL13B in replicate 2 and 3, and SPL9 and SPL2 in replicate 1 and 3 ( Fig. 3 ; Table 3 ; Supplementary Table S8 ). SPL13A and SPL13B are identical in open-reading frame, but differ in untranslated regions of their mRNAs. The similar expression correlations were also identified for miR172 and its target transcription factors; nearly all miR172 targets were downregulated, including SMZ in replicate 1 and 2, TOE1 in replicate 2 and 3, TOE2 in replicate 2 and SNZ in replicate 3, correlating with increased levels of miR172 ( Fig. 3 ; Table 3 ; Supplementary Table S8 ). The exception was also detected; TOE1 and TOE3 in replicate 1 were upregulated ( Fig. 3 ). Figure 3: The expressions in miR156 and miR172 targets regulated by CO 2 . Presented are CO 2 -regulated expression fold changes in miR156/157 and miR172 target transcripts of genes encoding SPL s and AP2- like transcription factors in three biological replicates, I, II, and III. The expression changes in SPL s and AP2 -like transcription factors were identified in RNA-seq experiments. Bars without colour represent SPLs ; numbers on these bars, 1, 2, 3, 4 and 5 represent SPL10, SPL9, SPL13A, SPL13B and SPL2 . Bars in grey colour represent AP2 -like transcription factors; numbers on the bars, 1, 2, 3, 4 and 5 are TOE1, SMZ, TOE3, TOE2 , and SNZ , respectively. The statistical tests were performed on transcript fold changes using Student’s t -test by comparing fragments per kilobase of transcript per million mapped reads or FPKM value (sample size) between samples, and the numbers are shown in Table 3 . Fold changes in target transcripts are statistically significant with P <0.01 (FDR test: q <0.1), or P <0.03 (FDR test: 0.1< q <0.2, marked by *). Full size image It was observed that Arabidopsis plants exposed to 810 p.p.m. [CO 2 ] flowered about 1 week earlier than those grown at 430 p.p.m. ( Fig. 1a ). This occurred without a change in leaf numbers. Our smRNA-seq and RNA-seq results indicated that this early-flowering phenotype was likely to be mediated by the miR156/miR157— SPLs —miR172— AP2-like transcription factor pathway ( Fig. 4a ). It is well-established that the sequential action of the components in this pathway controls the vegetative juvenile-to-adult phase transition and flowering time during normal development [29] . Specifically, miR156 is known to target and suppress the expressions of 10 SPL transcription factors, including SPL2 , − 3 , − 4 , − 5 , − 6 , − 9 , − 10 , − 11 , − 13 and − 15 (ref. 29 ). MiR157 shares 85.7% sequence identity with miR156, and both miRNAs suppress SPLs similarly [30] . MiR156 levels are at the highest in young seedlings and decline gradually over a period of several weeks into flowering development time ( Fig. 4a ) (ref. 31 ). When miR156 level is reduced, its target transcription factor, SPL9 , is upregulated, thus directly increases the transcription of miR172, which in turn suppresses AP2 and AP2 -like transcription factors such as TOE1 , TOE2 , TOE3 , SMZ and SNZ to promote adult epidermal identity and flowering ( Fig. 4 ) (refs 29 , 31 ). SPL9, −10, −2,− 3, −11, −13 and −15 have been shown to function similarly and redundantly with each other in regulation of the juvenile-to-adult phase transition and flowering time [29] , [30] , [31] , [32] , [33] , [34] , [35] , [36] . SPLs also feedback-regulate miR156 precursor transcription [29] . 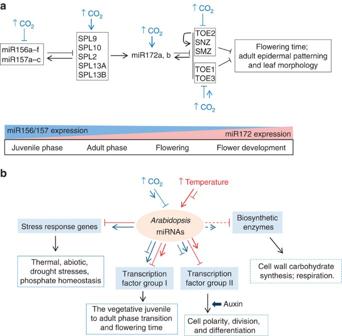Figure 4: Differentially expressed miRNAs in regulation of development. (a) The effects of elevated [CO2] on the expressions of miR156/157 and miR172 and their target transcriptional factors. These components function to regulateArabidopsisjuvenile-to-adult phase transition and flowering time. Shown below is a schematic diagram indicating the decline of miR156/157 and the rise of miR172 expression from the juvenile to the flowering development during plant development, adapted from Zhu and Helliwell50. SPLs, squamosa promoter binding protein-like transcription factors; AP2, APETALA2; TOE, TARGET OF EAT; SMZ, SCHLAFMUTZE; SNZ, SCHNARCHZAPFEN.↑CO2, elevated [CO2]. Blue arrows and stop signs represent promotion and suppression; black arrows and stop signs refer to promoting and suppressing actions during normal development. (b) The effects of elevated [CO2] and elevated temperature on miRNAs, the target genes of miRNAs, and their biological functions. Red colour, temperature regulated; blue colour, CO2regulated. ↑: upregulation; Τ, downregulation. The length of ↑ or Τ represents the relative numbers of miRNAs. The dash lines and boxes indicate the predicted results. The boxes with blue background contain miRNA target genes. Inside boxes with the blue outline are annotated functions of miRNA targets. The large black arrow indicates the auxin-mediated. Figure 4: Differentially expressed miRNAs in regulation of development. ( a ) The effects of elevated [CO 2 ] on the expressions of miR156/157 and miR172 and their target transcriptional factors. These components function to regulate Arabidopsis juvenile-to-adult phase transition and flowering time. Shown below is a schematic diagram indicating the decline of miR156/157 and the rise of miR172 expression from the juvenile to the flowering development during plant development, adapted from Zhu and Helliwell [50] . SPLs, squamosa promoter binding protein-like transcription factors; AP2, APETALA2; TOE, TARGET OF EAT; SMZ, SCHLAFMUTZE; SNZ, SCHNARCHZAPFEN.↑CO 2 , elevated [CO 2 ]. Blue arrows and stop signs represent promotion and suppression; black arrows and stop signs refer to promoting and suppressing actions during normal development. ( b ) The effects of elevated [CO 2 ] and elevated temperature on miRNAs, the target genes of miRNAs, and their biological functions. Red colour, temperature regulated; blue colour, CO 2 regulated. ↑: upregulation; Τ, downregulation. The length of ↑ or Τ represents the relative numbers of miRNAs. The dash lines and boxes indicate the predicted results. The boxes with blue background contain miRNA target genes. Inside boxes with the blue outline are annotated functions of miRNA targets. The large black arrow indicates the auxin-mediated. Full size image In summary, our results demonstrate that elevated [CO 2 ] has a significant impact on the miR156/157- SPLs -miR172- AP2s pathway likely through accelerating the normal decline of miR156/157 and the rise of miR172 during development. The correlated expression changes in SPLs and AP2s confirmed these effects, which could induce the early onset of flowering that was observed in the plants in response to elevated [CO 2 ]. Elevated temperature affects the miR156-regulated pathway We observed that a 3–5 °C increase in temperature advanced the flowering time in the plants by ~4–6 days ( Fig. 1b ). This was accompanied with fewer leaves, agreed with a previous report [5] . We showed that elevated temperature increased miR156/157 and decreased miR172 expressions, which is opposite to the effects of elevated CO 2 on these miRNAs ( Fig. 2b ; Supplementary Data 6 ). Inversely correlated expressions of miR156/157 targets were only identified in SPL2 , − 3 and − 13 in replicate 1, however, while SPL11 , −2 and −15 were expressed oppositely in replicate 1, 2 and 3, respectively ( Table 3 ). Mixed responses were also found in miR172 targets: TOE1 was downregulated by elevated temperature in replicate 1, while SMZ upregulated in replicate 2 ( Table 3 ). Our results demonstrate that elevated temperature can alter the expressions of all components in the miR156/157-SPLs-miR172-AP2s pathway in a complicated fashion. The role of this pathway played in regulating elevated temperature-induced early flowering needs to be further investigated. Elevated CO 2 and temperature affect miRNAs in auxin-signalling We identified five differentially regulated miRNAs that function in auxin-signalling pathways. MiR160, −167 and −390 target transcripts of auxin responsive factors ( ARFs ; Supplementary Table S9 ), which control auxin-regulated transcription. MiR164a–g and miR166a–g also target transcription factors and are involved in auxin-regulated organ development ( Supplementary Table S9 ). A strong expression correlation was identified between miR164 and its targets, NAC family members; NAC1 was downregulated by elevated temperature in two biological replicates, correlated inversely with miR164 expression ( Fig. 2c ; Table 3 ; Supplementary Table S8 ). NAC1 is required for transducing auxin signals for lateral root emergency and the development of embryonic, leaves and floral organs ( Supplementary Table S9 ). Another expression correlation example is related to miR160. Normally, miR160 negatively regulates the expressions of ARF10 , −16 and −17 , which promote cell divisions in a variety of tissues ( Supplementary Table S9 ). Elevated temperature downregulates ARF17 , while elevated [CO 2 ] upregulates ARF10 ; both correlated inversely with miR160 expression ( Fig. 2a,b ; Table 3 ; Supplementary Table S8 ). Thus, elevated temperature might reduce plant growth through down- and upregulating the expressions of miR164 and miR160, respectively, while elevated [CO 2 ] may enhance it through decreasing miR160. Elevated CO 2 and temperature affect stress-responsive miRNAs Expressions of six stress-responsive miRNAs were altered significantly by elevated [CO 2 ] and/or elevated temperature ( Fig. 2a–c ). The inversely correlated expression was detected between miR162 and its target, dicer-like 1 transcript in one biological replicate ( Table 3 ; Supplementary Table S8 ). The expression changes in miR162 and its target have been demonstrated previously to be induced by drought, cold and salt ( Supplementary Table S9 ). However, the targets of miR161.1, −169, −158, −399 and −5026 were not found with significant expression changes ( Supplementary Table S9 ; Supplementary Data 15,16 ). Predicted target genes of new miRNAs Using the psRNATarget webserver [37] and Degradome data [28] , we predicted targets of differentially regulated new miRNAs ( Supplementary Methods ; Table 2 ; Supplementary Data 17 ). Several of these targets have previously annotated functions ( Table 2 ). For example, miRPAL2 target, galacturonosyltransferase-like 9 ( GATL9 ) or glucosyl transferase family 8 ( LGT8 ) gene functions in cell wall pectin and/or xylan biosynthesis [38] . MiRPAL5 targets the transcripts of cellulose synthase 10 (ref. 39 ), a member in cellulose synthase family that catalyses the reaction between substrates, uridine diphosphate glucose and a chain of 1,4-beta- D -glucosyl residues to generate uridine diphosphate and an elongated chain of glucosyl residues or cellulose ( Table 3 ; Supplementary Data 17 ). The predicted target gene of miRPAL3, nudix hydrolases 11 ( Table 3 ; Supplementary Data 17 ) encodes a protein that has pyrophosphatase activity with CoA as its substrate [40] . None of the predicted miRNAs were found with significant expression changes in their target genes except miRPAL2 ( Table 3 ; Supplementary Table S8 ). As these miRNAs all expressed lowly, it is unclear whether their expression changes can lead to phenotypic changes. Using deep-sequencing methods, we identified known and predicted miRNAs that were regulated differentially by elevated [CO 2 ] and/or elevated temperature. We categorized these miRNAs into four groups based on the annotated functions of their targets as follows ( Fig. 4b ): Group I targets the transcription factors that control Arabidopsis juvenile-to-adult phase transition and flowering time; Group II targets the transcription factors that regulate auxin-mediated cell polarity, division and differentiation during Arabidopsis development; Group III targets the stress-responsive genes; Group IV includes newly predicted miRNAs that target potentially genes involved in cell wall carbohydrate synthesis, respiration and other functions. The sequential action of Group I miRNAs, miR156/157 and miR172 control vegetative traits and the transitional timing from vegetative to reproductive phase during development [29] . Manipulations of the expression in these miRNAs can change Arabidopsis flowering time; for example, the overexpression of miR156 prolongs the juvenile phase and delays flowering time [29] , [34] , [41] , while its reduction is similar to SPLs overexpression, leading to the early-flowering phenotype [29] , [42] . Overexpressed miR172 also results in the early-flowering phenotype [29] , [43] . In this study, we identified the correlated expression changes in all components in this pathway with the fold changes of 0.37–0.85 and 0.63–0.80 in miR156a–f and miR157a–c, 1.44–2.40 in miR156 targets, SPLs , 1.40–2.19 in miR172a, b and 0.14–0.67 in miR172 targets, AP2s (except two targets in Biological replicate 1) in elevated CO 2 -treated 10-leaf stage leaves ( Fig. 2a ; Fig. 3 ; Supplementary Table S8 ). These are comparable changes to development-driven expressions: 0.3- and 2.4-fold changes were observed in miR156 and miR172 between 12 and 26 days of plants (short day) [29] , thus might be sufficient to induce early flowering. The potential difference in development between 10-leaf stage leaves treated by different [CO 2 ], if there is any at all, is unlikely to result in the expression changes that can be reached in many days during development. The correlated expressions in miR156/157 and miR172 targets, SPLs and AP2s support that this pathway was indeed affected by a high level of [CO 2 ]. The significant downregulation in miR172 targets, AP2s seems unusual as AP2s do not respond to miR172 expression significantly during development [44] , [45] . It has been proposed that miR172 regulation of its targets is a balanced result of translation suppression [44] , [45] , transcript cleavage [43] , [44] , [46] , [47] and self-feedback regulation [47] of these targets [46] . A recent study showed that this balance may be changed under stress; it was found that miR172 targets, SMZ and TOE2 increased significantly in expression at 16 °C, correlating with a significant decrease in miR172 (ref. 22 ). Therefore, it is likely for significant decreases in miR172 targets under high [CO 2 ] stress to occur. We do not know how elevated [CO 2 ] affects the miR156/157-SPLs-miR172-AP2s pathway, whether through acting on miR156 expression alone, which, in turn, alters sequentially the expressions in its downstream components, or by effecting all components independently ( Fig. 4a ). Given that these components regulate with each other either directly or through feedback loops, it is hard for the correlated expression changes to occur coincidently. The advantage of sequencing is that an expression profile of miRNAs and mRNAs involved in all biological pathways or networks can be generated at the same time. The information generated can be highly valuable, considering that expression levels are crucial for the silencing effects of miRNAs and the function of mRNAs, particularly to those miRNAs and their targets that are known to regulate-specific phenotypes. Nevertheless sequencing approach does not provide the details on how CO 2 act to affect this pathway, directly or indirectly. This information can be only obtained through genetic analysis. To understand whether other flowering regulatory genes contribute to the early-flowering time induced by elevated [CO 2 ] and temperature, we examined the expressions of some early markers of flower development including SOC1, FRUITFUL (FUL), AP1, CAULIFLOWER (CAL), LEAFY (LFY) and some floral transition genes, FLC , FLOWER LOCUS M (FLM) , FLOWER LOCUS T (FT) , CONSTANS (CO) and LONG DAY (LD) [48] in our RNA-seq data. For CO 2 -treated samples, we detected the increased expressions in FT and FUL in two biological replicates ( Supplementary Data 15 ). FT and FUL promote the onset of flowering, and AP2s antagonize their expressions [49] , suggesting that the downregulation of AP2s by elevated [CO 2 ] can promote flowering potentially through upregulating FT and FUL . However, we cannot exclude completely the involvement of other flowering regulatory genes until other developmental time points are also investigated and genetic studies are conducted. In temperature-treated samples, we detected significant expression differences in several flowering regulatory genes including GI , FT , FLM , FLC and AP1 , but not GIGANTEA ( GI ) and SHORT VEGETATIVE PHASE ( SVP ) that controls the expression of miR172 ( Supplementary Data 16 ) (refs 50 , 51 ). A 4.2-fold increase in FLC and a ~1.8-fold decrease in FLM support a previous finding that FLC potently suppressed thermal induction, while the closely related floral repressor, FLM , was a major-effect quantitative trait locus modulating thermo-sensitivity [4] . These results suggest that the miR156-regulated pathway might play a minor role in thermo-induced early flowering. None of our identified miRNAs target the transcripts of proteins involved directly in light and dark reactions of photosynthesis and photorespiration [52] . Nevertheless, elevated sugar levels in leaf tissues resulting from enhanced photosynthesis by elevated [CO 2 ] have been shown to affect plant metabolism, development and gene expression [53] . It was hypothesized that sugar can affect the developmental transitions and are highly responsive to environmental signals [53] . For example, 1% sucrose was reported to promote floral transition of late-flowering mutants [54] . This suggests that elevated [CO 2 ] might induce the early flowering by increased sugar level. It has also been shown that hexoses tend to affect cell division and expansion, whereas sucrose favors differentiation and maturation [53] . It will be interesting to see whether sugar affect miRNAs in flowering- and auxin-signalling pathways. Microarray studies revealed the expression changes in homologues of the genes affected by CO 2 (refs 11 , 12 , 13 , 14 , 15 , 16 ). In C. reinhardtii, elevated [CO 2 ] downregulated the expressions of five SPLs , although in the opposite direction of that observed in this study [15] . In sugarcane, ARF2 was found to be downregulated, suggesting that auxin-signalling is also involved [14] . We did not find the conservation of miRNA targets in poplar [13] and soybean [16] , perhaps because only a proportion of total genes were analysed in these species. In our RNA-seq results, not all targets of miR156/157 and miR172 were found to be altered differentially, and the differentially regulated targets were not identified in the same biological replicates. This nonselective targeting might be contributed by multiple factors such as miRNA expressions, expression patterns of miRNA target genes, the accessibility of target sites by miRNAs, and feedback regulation of miRNAs by target transcripts [55] . A previous study demonstrated that multiple mRNAs could be successfully targeted by artificially designed miRNAs, but the degree of downregulation varied for different targets [55] . It was shown that no clear correlation of targeting efficiency was found either with the extent of complementarity between artificial miRNAs and targets or with expression levels of targets [55] . In addition, RNA-seq technique has been shown recently with technical variability particularly in exons at low levels of read coverage, and the relative abundance of a transcript can also substantially disagree [56] . Besides, plant intrinsic variations might contribute to the variations in miRNA expressions, which exhibited as opposite or subtle expression changes compared with the majority, particularly in response to low levels of environmental changes, that is , 26 o C temperature. The intrinsic variation is readily observed during plant development; for example, flowering time may vary in a few days in plants grown from the seeds descended from the same plant. In this study, we showed that Arabidopsis seed and biomass production were both significantly increased by elevated [CO 2 ], but decreased by elevated temperature ( Fig. 5 ). As nearly all elevated CO 2 -regulated miRNAs were inversely regulated in expression by elevated temperature, it is likely for those that function to regulate plant growth to contribute to the opposing effects of elevated [CO 2 ] and elevated temperature on plant biomass and seed production. Further investigations on individual miRNAs will help us to elucidate their roles in plant yields. 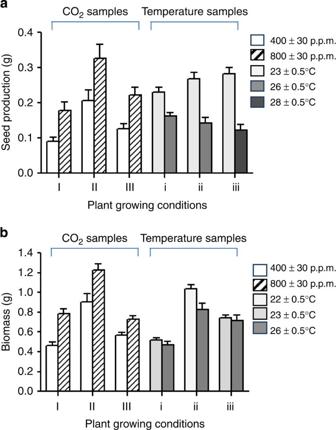Figure 5: The opposing effects of CO2and temperature onArabidopsisyield. Shown in this figure are (a), seed and (b), biomass production in three independently grown plants under different [CO2] and different temperatures. All sample pairs are different statistically between the control and the testing condition by Student’st-test (P<0.05), except one temperature pair marked by *. For seed production, the number of plants used:n=9, 8, and 9 for 400 p.p.m.- andn=9, 9, and 9 for 800 p.p.m.-treated samples;n=10, 11, and 7 for 23 °C- andn=8, 11, and 6 for 26–28 °C-treated samples. For biomass production, the number of plants used:n=8, 8, and 10 for 400 p.p.m.- andn=8, 8 and 9 for 800 p.p.m.-treated samples;n=10, 9, and 7 for 23 °C- andn=8, 8, and 6 for 26–28 °C-treated samples. For CO2-treated plants, seeds and above-ground biomass were collected in two months of plant growth in biological replicate II, and 2 weeks earlier in replicate I and III. Biomasses do not include the weights of collected seeds. Figure 5: The opposing effects of CO 2 and temperature on Arabidopsis yield. Shown in this figure are ( a ), seed and ( b ), biomass production in three independently grown plants under different [CO 2 ] and different temperatures. All sample pairs are different statistically between the control and the testing condition by Student’s t -test ( P <0.05), except one temperature pair marked by *. For seed production, the number of plants used: n =9, 8, and 9 for 400 p.p.m.- and n =9, 9, and 9 for 800 p.p.m.-treated samples; n =10, 11, and 7 for 23 °C- and n =8, 11, and 6 for 26–28 °C-treated samples. For biomass production, the number of plants used: n =8, 8, and 10 for 400 p.p.m.- and n =8, 8 and 9 for 800 p.p.m.-treated samples; n =10, 9, and 7 for 23 °C- and n =8, 8, and 6 for 26–28 °C-treated samples. For CO 2 -treated plants, seeds and above-ground biomass were collected in two months of plant growth in biological replicate II, and 2 weeks earlier in replicate I and III. Biomasses do not include the weights of collected seeds. Full size image In summary, we identified known and predicted miRNAs, their target genes and molecular pathways that are regulated by elevated [CO 2 ] and elevated temperature. Our results demonstrate that the miR156/157- SPLs -miR172- AP2-like transcription factor pathway is likely to have a major role in elevated [CO 2 ]-induced early flowering. The conservation of this pathway in plant species suggests its fundamental role in controlling plant flowering time in response to increasing atmospheric CO 2 concentration. Both CO 2 and temperature can also regulate miRNAs and their targets in several pathways, which modulate plant growth and development. The opposing effects of these two conditions on several miRNAs suggest mechanistic clues for understanding the interactions of CO 2 and temperature in regulation of plant growth and development. Our results have opened new perspectives for understanding plant response and adaptation to climate change. Arabidopsis plant growth conditions Seeds of Arabidopsis thaliana (ecotype Col-0) were imbibed at 4 °C with distilled water for 4 days to facilitate uniform germination. The seeds were resuspended in 0.05% agarose after the cold treatment and planted in 1m 3 mesocosms in greenhouse where low (430±50 μmol mol −1 or p.p.m.) and high (810±50 μmol mol −1 or p.p.m.) carbon dioxide concentrations were maintained and monitored every hour daily. The temperature was set between 24 °C and 18 °C (the highest during the day/the lowest at night), natural lighting was augmented on overcast days with sodium halide lamps, and humidity was maintained at natural conditions. All environmental parameters were monitored every hour daily. After five self-seeding generations, the sixth generation plants were grown for this study. The plants grown under 810 p.p.m. [CO 2 ] were seen the first inflorescence stems on the 70th day after plant germination and those under 430 p.p.m. concentration a week later ( Fig. 1a ). The onset of flowering in these plants occurred within 5–6 weeks. A sample consisting of a pool of 100 uppermost fully expanded rosette leaves from plants at the 10 leaves stage were chosen and collected at random from the mesocosm population using a point-grid system. Samples grown under 810 and 430 p.p.m. [CO 2 ] were collected at the same time, about 1 or 2 weeks before first inflorescence stems were observed, respectively ( Fig. 1a ). Leaves were sampled onto liquid nitrogen and stored at −80 °C until further analysis. Although 400 and 800 p.p.m. were CO 2 concentrations to be obtained, our calculation of means based on all recorded [CO 2 ] concentrations during plant growth indicate the mean values as 430 and 810 p.p.m. To grow plants at different temperatures, Arabidopsis seeds (ecotype Col-0) were soaked in water and then planted onto soils (Cat no. : 65-3191; Sunshine LC1 Suncoir Mix) that were previously wet in KORD 3.0 Sq Grn 504 growing pots (Cat no. : 50-1210; Griffin Greenhouse and Nursery Supplies Inc.). The growing pots were then moved into a 4 °C cold room for 3 days before being transferred into two GCW30 Arabidopsis walking-in chambers (Environmental Growth Chambers Inc.) set with 22±0.5 and 28±0.5 °C and long-day lightening (16 h light/8 h dark). Plants used for stem-loop real-time PCR verification experiments were grown in an Arabidopsis growth chamber with two identical and independent units (AR22L; Percival Inc.). Uppermost fully expanded rosette leaves were collected from 8–10 plants with 1–2 inches stems at bolting stage grown under different temperature conditions; plants grown at 26 or 28 °C were collected about 4 or 6 days earlier than those grown at 22 or 23 °C ( Fig. 1b ). Collected leaves were frozen immediately in liquid nitrogen for storage. Two pairs of samples grown at 430 and 810 p.p.m. [CO 2 ], and one pair at 22 and 28 °C temperatures were used to extract total RNAs in preparation of smRNA libraries for sequencing. Seed and biomass production under different levels of temperatures and [CO 2 ] were analysed in plants grown in Arabidopsis growth chambers (AR22L; Percival Inc.). The plant growing conditions included long-day lightening (16 h light/8 h dark) and 65% humidity and optimum lightening condition. The temperatures were the same as described above, and CO 2 concentrations were 400±30 and 800±30 p.p.m. Seeds were collected from plants grown up to 2 months, except those CO 2 -treated plants in I and II ( Fig. 5 ) for 1 month and a half. For plant biomass production, above-ground plants were collected and dried in 55 o C oven for 1 week, and weighted. Preparation of smRNA-seq and RNA-seq libraries Total RNAs were extracted from frozen leaves using TRIzol Reagent (Life Technologies Cat no. 15596-026). The smRNA libraries were prepared using a Digital Gene Expression for Small RNA Sample Prep Kit purchased from Illumina Inc. (P/N: 1002398) following the manufacturer’s instructions. These libraries were then sequenced on Illumina Genome Analyzer IIx (GAIIx) Sequencer. For generating RNA-seq libraries, total RNAs were extracted similarly as described above. The qualities of total RNAs were checked with 2100 Bioanalyzer (Agilent Inc.), and those that have good quality were used for making RNA-seq libraries. RNA-seq libraries were prepared using TruSeq RNA Sample Preparation v2 kit (Illumina Inc.) following manufacturer’s instruction. The qualities of the libraries were analysed with Bioanalyzer before sequencing on Illumina Hi-seq2000 Sequencer. Sequencing data was deposited under the National Gene Expression Omnibus series number, GSE36934 . General analyses of smRNA-sequencing data The smRNA reads from all libraries were 3′ trimmed using NOVOALIGN ( http://www.novocraft.com ). Reads containing low complexity regions such as poly (A) stretches and low quality reads (containing N’s) were removed, and filtered for length 15–30 nts. All read sets from the different conditions were subsequently mapped onto the Arabidopsis TAIR9 genome and data set sequences using RazerS [57] . Known miRNA reads were obtained by matching mapped reads to annotated miRNAs with no mismatch. For annotating isomirs and miR-siblings for known miRNAs, we used mapped reads without mismatch in sense direction onto miRNA precursor sequences annotated in miRBase16, which have a minimum abundance of 20 reads, but do not represent annotated miRNA mature and star sequences. We defined isomirs as reads that are not shifted >5 positions from their original mature or star 5′-position and miR-siblings as the remaining highly abundant reads that were mapped to the miRNA precursor. Reads mapping to annotated transcripts or regions were normalized as reads per million per library. The prediction of new miRNAs For prediction of new miRNAs, reads matching with no mismatch to TAIR9 cDNA, annotated miRNA, tRNA, snoRNA or other non-coding RNA sequences were removed from mapped reads ( Supplementary Table S1 ). For each condition, reads with a minimum abundance of 20 reads and fewer than 25 distinct matches on the TAIR9 genome were collected for further processing. Two distinct strategies were used to detect hitherto unknown miRNAs: miRCat [24] and an in-house plant-specific version of miRDeep ( Supplementary Methods ) [25] , [26] , [58] . A workflow is presented in Supplementary Fig. S2 , and read analyses are summarized in Supplementary Table S1 . The determination of differentially expressed miRNAs All predicted and miRBase 16 annotated miRNAs were analysed to detect differential expression between corresponding conditions (430 versus 810 p.p.m., and 22±0.5 °C versus 28±0.5 °C) using the χ 2 -test for P -value calculation and the Benjamini-Hochberg method for multiple-testing correction (false discovery rate (FDR) q <0.05) as described previously [59] . The biological replicates for the CO 2 experiments showed a high correlation in normalized miRNA reads (Spearman's rank correlation rho of 0.94 and 0.89 for 430 and 810 p.p.m., respectively). To determine the differential expressions of each miRNA family, we tallied the counts for each of its mature sequences, then star, and finally the most abundant. A χ 2 -test ( P <0.01) was applied using normalized counts in temperatures and CO 2 conditions versus the total read counts for each library. P -values were adjusted using the Benjamini-Hochberg method for calculating FDR ( q <0.05). The determinations of differentially expressed miRNA targets The RNA-seq analysis was performed using GALAXY online tools. The raw RNA-seq reads were mapped uniquely to Arabidopsis Tair10 reference genome by TopHat (paired-end). Gene model was downloaded from ftp://ftp.arabidopsis.org/home/tair/Genes/TAIR10_genome_release/ . Cufflinks was used to assemble transcripts and estimate the abundances, and Cuffcompare to compare the assembled transcripts to reference annotation. A list of differentially expressed genes was obtained by applying Cuffdiff between two samples in each biological replicate. Both Cufflinks and Cuffdiff used upper-quantile normalization to normalize total mapped reads. Expression read normalization was done between two samples in each replicate, but not among all three pairs of samples. Transcripts that overlapped with differentially expressed genes were then identified by genome locations. The potential targets of newly predicted mature miRNAs that are differentially regulated were predicted using the psRNATarget webserver [37] at http://plantgrn.noble.org/psRNATarget/ with the TAIR9 annotated transcripts as potential target sequences. Quantification of miRNAs by Taqman stem-loop RT–qPCR Taqman stem-loop RT–qPCR reactions were performed to quantify known miRNAs following previously published method [23] and manufacturer’s instructions (Applied Biosystem Inc.). To quantify predicted miRNAs, we designed stem-loop RT primers and qPCR primers based on previously published method ( Supplementary Data 18 ) (ref. 60 ), and SYBR Green was used in qPCR reactions. Expression fold changes for each miRNA between different CO 2 concentrations- or different temperatures-treated samples ( Supplementary Data 5, 6, 13, 14 ) were calculated as follows: Ct: Cycle threshold. Ct 5s rRNA : Ct number obtained for the internal control 5s rRNA. −ΔΔ T : −[(Ct higher temperature sample −Ct higher temperature 5s rRNA )−(Ct lower temperature sample −Ct lower temperature 5s rRNA )]. −ΔΔ C : −[(Ct higher CO2 concentration sample −Ct higher CO2 concentration 5s rRNA ) − (Ct lower CO2 concentration sample −Ct lower CO2 concentration 5s rRNA )]. Expression fold changes were obtained by calculating antilog 2 (–ΔΔ). The statistical significance was obtained for miRNAs that showed the same expression trend for at least four times by χ 2 -test, P <0.05. Accession codes: Sequencing data can be found under National Center for Biotechnology Information Gene Expression Omnibus series number, GSE36934 .Contact: Patrick May, Qiong A. Liu. How to cite this article: May, P. et al. The effects of carbon dioxide and temperature on microRNA expression in Arabidopsis development. Nat. Commun. 4:2145 doi: 10.1038/ncomms3145 (2013).